Small RNA changesen routeto distinct cellular states of induced pluripotency MicroRNAs (miRNAs) are critical to somatic cell reprogramming into induced pluripotent stem cells (iPSCs), however, exactly how miRNA expression changes support the transition to pluripotency requires further investigation. Here we use a murine secondary reprogramming system to sample cellular trajectories towards iPSCs or a novel pluripotent ‘F-class’ state and perform small RNA sequencing. We detect sweeping changes in an early and a late wave, revealing that distinct miRNA milieus characterize alternate states of pluripotency. miRNA isoform expression is common but surprisingly varies little between cell states. Referencing other omic data sets generated in parallel, we find that miRNA expression is changed through transcriptional and post-transcriptional mechanisms. miRNA transcription is commonly regulated by dynamic histone modification, while DNA methylation/demethylation consolidates these changes at multiple loci. Importantly, our results suggest that a novel subset of distinctly expressed miRNAs supports pluripotency in the F-class state, substituting for miRNAs that serve such roles in iPSCs. Reprogramming of somatic cells into induced pluripotent stem cells (iPSCs), by forced expression of the transcription factors Oct4, Sox2, Klf4 and c-Myc (OSKM), entails a dramatic transformation of their gene expression programme and a resetting of their epigenetic state [1] , [2] . iPSCs have transcriptome and epigenome characteristics similar to embryonic stem cells (ESCs), the ‘gold standard’ of pluripotency. Given the promise that lies in applying iPSC-based approaches in drug discovery and regenerative medicine there is great interest in more fully understanding the molecular basis of, and the reprogramming routes that lead to, pluripotency. Forming an international alliance to address these issues we explored alternative outcomes of somatic reprogramming and discovered an alternate stable pluripotent state represented by a class of fuzzy colony forming cell lines (F-class) that can arise when OSKM expression is maintained at high level [3] . To model time-resolved molecular trajectories of somatic cell reprogramming towards the F-class and ESC-like states, we used doxycycline-inducible OSKM expression in secondary murine embryonic fibroblasts (2°MEFs) [4] . Multiple global data sets were acquired in parallel, ranging from epigenomics to transcriptomics and proteomics, each concordantly describing the progression of cells to either a classic ESC-like state or the novel F-class state [4] , [5] , [6] . These data sets are available through http://stemformatics.org [7] , and form a unique resource to further pluripotency research. The expression of multiple miRNAs is altered during reprogramming [8] , [9] , [10] . miRNAs furthermore play a critical role in the process, as transcription factor-driven reprogramming can be enhanced or replaced by the expression of specific subsets of miRNAs known to be highly expressed in iPSCs [11] , [12] . Here we use next generation sequencing (NGS) to analyze small RNA expression at nucleotide resolution as 2°MEFs transition towards distinct pluripotent states. We observe widespread changes, often characteristic of either the ESC-like or F-class state. Gene ontology (GO) enrichment analysis of experimentally validated targets of co-clustered miRNAs revealed complex temporal regulation of cell growth, viability, morphology and underlying molecular processes throughout reprogramming. Drawing on the genome-wide epigenome and long RNA transcriptome data sets acquired in parallel provides vistas into intricate multi-level control of miRNA expression. Time-resolved small RNA sequencing of 2°MEF reprogramming We used doxycycline-inducible OSKM expression in 2°MEFs [4] to establish cell cultures that transitioned to distinct pluripotent states, by branching the doxycycline concentration in the media at day 8. Keeping doxycycline level at 1,500 ng ml −1 (high OSKM) led to the F-class state, while decreasing it to 5 ng ml −1 (low OSKM) led to the ESC-like state. We sampled the process at the time points indicated in Fig. 1a (sample nomenclature, for example, D8 H: day 8, high OSKM), while 1°iPSCs, 2°iPSCs [4] and Rosa26-rtTA knock-in ESCs [4] served as ESC-like controls (See Methods and Supplementary Data 1 for details). Small RNA library composition shifted away from miRNAs during reprogramming, from ~79% of tags representing miRNAs in 2°MEFs to a low of ~42% in D16 H; during low OSKM reprogramming this proportion approached the level of ~65% observed in ESC-like controls ( Fig. 1b , Supplementary Fig. 1a ). Nevertheless, quantitative PCR (qPCR) analyses demonstrated that levels of a set of indicator miRNAs remained relatively steady across samples ( Fig. 1c ). The proportion of tags mapping to the nuclear genome outside annotated miRNA loci increased from ~20% in 2°MEFs to as high as ~42% in D16 H ( Fig. 1b ); these tags displayed a range of lengths, expression patterns and mapped to multiple distinct loci categories ( Supplementary Fig. 1b,e ). Tags mapping to the mitochondrial (mt) genome also varied in length ( Supplementary Fig. 1c ) and, interestingly, their proportion differed markedly between 2°MEFs (~1%), F-class cells (~16% in D16H) and ESC-like controls (~4%) ( Fig. 1b , Supplementary Fig. 1e ). mt-DNA-mapped tags were primarily associated with certain transfer RNA genes but also the D-loop control region, as reported [13] ( Supplementary Fig. 2 ). A locus immediately downstream of mt-transfer RNA MT-TV accounted for much of the change in library proportion, as validated by qPCR ( Fig. 1c ). Other small RNA species derived from a variety of nuclear and mt-DNA loci also increased in abundance, particularly towards the F-class state, likely reflecting opening of chromatin followed by consolidation into the distinct epigenetic states of F-class and ESC-like cells [4] , as well as changes in mitochondrial function and increased proliferation during reprogramming [5] , [14] , [15] . Altogether, in a background of dramatic small RNA changes, reprogramming cells retained miRNA pools of similar size relative to total RNA content, highlighting the importance of tight regulation of miRNA levels. 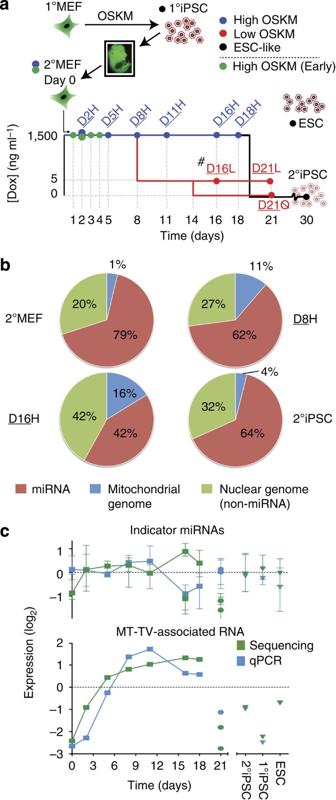Figure 1: Features of small RNA expression during secondary reprogramming. (a) Outline of doxycycline-inducible secondary reprogramming system (1B4and sampling strategy. Samples (n=1): high OSKM (blue), low OSKM (red), ESC-like controls (black) and (re)sequencing of early samples (green).#OSKM transgene expression was partially silenced inD6L cells, but was almost completely abolished in D21L and D21cultures3. (b) Small RNA libraries were analyzed to an average depth of ~27 million genome-mapped tags per sample. Tags distributed across diverse genomic loci, shown here for representative samples. (c) Top: miR-191, -484, -16, -149 and -30e were chosen from NGS data for their relatively stable expression across samples and validated by qPCR (averaged expression of all five miRNAs is shown, bars represent expression range). Bottom: expression of an abundant small RNA mapping to an mt-DNA region 3′ of mt-transfer RNA-V was measured by NGS and qPCR. NGS data were normalized to mapped tags, qPCR results were first normalized to total RNA input and then to average expression across all samples. Figure 1: Features of small RNA expression during secondary reprogramming. ( a ) Outline of doxycycline-inducible secondary reprogramming system (1B [4] and sampling strategy. Samples ( n =1): high OSKM (blue), low OSKM (red), ESC-like controls (black) and (re)sequencing of early samples (green). # OSKM transgene expression was partially silenced in D6 L cells, but was almost completely abolished in D21L and D21 cultures [3] . ( b ) Small RNA libraries were analyzed to an average depth of ~27 million genome-mapped tags per sample. Tags distributed across diverse genomic loci, shown here for representative samples. ( c ) Top: miR-191, -484, -16, -149 and -30e were chosen from NGS data for their relatively stable expression across samples and validated by qPCR (averaged expression of all five miRNAs is shown, bars represent expression range). Bottom: expression of an abundant small RNA mapping to an mt-DNA region 3′ of mt-transfer RNA-V was measured by NGS and qPCR. NGS data were normalized to mapped tags, qPCR results were first normalized to total RNA input and then to average expression across all samples. Full size image miRNA processing and expression dynamics As expected, miRNA-mapped tags had a sharp modal length of 22 nt ( Supplementary Fig. 1d ), and a small number of abundant miRNAs dominated the tag count (for example, the top 10 miRNAs represented ~50% of tags; Supplementary Data 1 ). miRNA processing variants can have alternative messenger RNA (mRNA) targeting properties and their relative proportions have been shown to alter between tissues and during development [16] . miRNA processing diversity was evident throughout reprogramming at proportions similar to other cell types [17] , [18] ( Fig. 2 ; Supplementary Fig. 3 ; detailed views of these parameters, generated with the miRSpring tool [19] are provided in Supplementary Data 3–15 ). Many pluripotency-related miRNAs were expressed as multiple isoforms, which presents important implications for their biological function and reliable detection. For example, 19/24 miRNAs encoded by the miR-290-295 and miR-302/367 loci co-expressed multiple isoforms (11 with 5′ isomiRs, 14 with 3′ isomiRs and 2 with non-templated addition), and 5/12 hairpins had appreciable expression from both arms ( Supplementary Figs 4 and 5 ). Surprisingly, we saw little directional isoform variation along reprogramming trajectories (including non-templated additions) and thus widespread changes in miRNA processing bias are not a feature of this process ( Supplementary Fig. 3 ). By contrast, even though bulk miRNA levels remained stable, expression levels of most individual miRNAs changed dramatically during reprogramming and we confirmed these changes for 17 examples by qPCR analyses ( Supplementary Figs 6 and 7 ). Principal component ( Fig. 3a ) and Pearson correlation analyses [4] of miRNA expression demonstrated that cells on the high OSKM trajectory reprogrammed towards the stable F-class state, while those on the low OSKM trajectory approached characteristics of ESC-like controls. 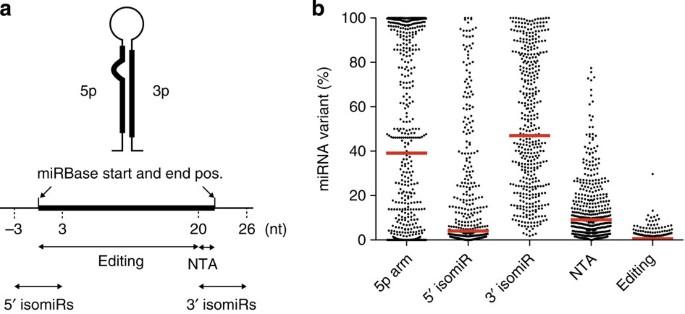Figure 2: miRNA processing variants. (a) Simplified schematic of the types of variants enumerated inb. (b) Scatter dot plot showing the average contribution of processing variants to miRNA expression across 13 samples represented inFig. 1aas red, blue and black circles. Red line represents median variant proportion across all microRNAs. Graphs display data for 424 miRNAs, thresholded for an average expression of >25 counts per million (CPM) per sample. Figure 2: miRNA processing variants. ( a ) Simplified schematic of the types of variants enumerated in b . ( b ) Scatter dot plot showing the average contribution of processing variants to miRNA expression across 13 samples represented in Fig. 1a as red, blue and black circles. Red line represents median variant proportion across all microRNAs. Graphs display data for 424 miRNAs, thresholded for an average expression of >25 counts per million (CPM) per sample. 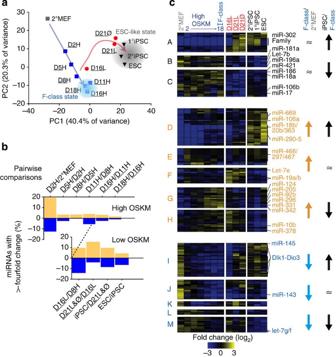Figure 3: miRNA expression dynamics in reprogramming cell states. (a) Principal component projection plot for miRNA profiles. Samples: 2°MEFs (grey square), high OSKM (blue squares), low OSKM (red circles) and ESC-like controls (black triangles). Arrows indicate distinct sample trajectories. (b) Percentage of differentially expressed miRNAs (>fourfold) between successive time points (upregulated, yellow; downregulated, blue). (c) miRNA expression was normalized to average expression in all samples, and profiles were clustered as detailed inSupplementary Fig. 7. Shown here is a subset of clusters further categorized based on expression in the high OSKM trajectory and ESC-like cells. Profiles of selected miRNAs are indicated on the right. Analyses included 217 miRNAs that were within the top 95th percentile of expression in at least one sample. Full size image Figure 3: miRNA expression dynamics in reprogramming cell states. ( a ) Principal component projection plot for miRNA profiles. Samples: 2°MEFs (grey square), high OSKM (blue squares), low OSKM (red circles) and ESC-like controls (black triangles). Arrows indicate distinct sample trajectories. ( b ) Percentage of differentially expressed miRNAs (>fourfold) between successive time points (upregulated, yellow; downregulated, blue). ( c ) miRNA expression was normalized to average expression in all samples, and profiles were clustered as detailed in Supplementary Fig. 7 . Shown here is a subset of clusters further categorized based on expression in the high OSKM trajectory and ESC-like cells. Profiles of selected miRNAs are indicated on the right. Analyses included 217 miRNAs that were within the top 95th percentile of expression in at least one sample. Full size image An early and a late wave of pronounced change to epigenetic, transcriptomic and proteomic profiles has been reported during reprogramming [1] , [4] , [8] , [15] . We observed that miRNA expression changes featured two distinct bursts, one within 48 h of transgene expression (for example, 43/132 of appreciably expressed miRNA change more than fourfold) and the second burst beyond day 8, notably more pronounced in the low OSKM trajectory ( D11 H/ D8 H: 14/135; D16 L/ D8 H: 34/138; Fig. 3b ). Sampling the early stages of reprogramming (2°MEF E , D1 H E , D2 H E , D3 H E , D4 H E ) indicated that 20/134 appreciably expressed miRNAs changed more than fourfold within the first 24 h ( Supplementary Fig. 8a,b and Supplementary Data 16–21 ). Hierarchical clustering ( Fig. 3c ; Supplementary Figs 7a and 8c ) and GO enrichment analysis of experimentally validated targets of co-clustered miRNAs ( Supplementary Figs 7b and 8d ) revealed that processes important during reprogramming, such as cell cycle/proliferation, apoptosis, cell morphology, development/differentiation, signal transduction and gene regulation through chromatin modification, transcription and RNA processing, were all targeted by complex temporal patterns of miRNA change. Notably, even though the majority of miRNA expression clusters ( Fig. 3c , clusters A-D, G-I, L, M) indicated pronounced differences between the F-class and ESC-like state, these distinct subsets of miRNAs targeted similar cellular processes throughout both reprogramming trajectories. Multi-level control of miRNA expression Drawing on the genome-wide epigenome and long RNA transcriptome data sets acquired in parallel [4] , [5] , [6] we annotated 71 loci (representing 128 mature miRNA) with available data for pri-miRNA expression, as well as promoter DNA (CpG) methylation and histone lysine trimethylation (activating H3K4me3 and repressing H3K27me3; Supplementary Fig. 9 ). Overall, mature and pri-miRNA expression levels were moderately well-correlated across samples, with a higher correlation at early time points indicative of strong transcriptional control of miRNAs in the first few days after OSKM induction. Dividing miRNAs into those derived from intragenic or intergenic loci revealed a better correlation with pri-miRNA expression for the latter, highlighting a need for uncoupling of intragenic miRNA regulation from host gene expression ( Fig. 4a , supported also by histone trimethylation shown in Fig. 4b,c ). Fifteen, mostly intragenic miRNA loci with the poorest miRNA/pri-miRNA correlation were selected for closer inspection ( Supplementary Fig. 10 ). Evidence of complex or novel promoter usage explained this poor correlation for four loci, while the remaining loci are strong candidates for regulation at the post-transcriptional level (that is, through affecting miRNA processing or stability). 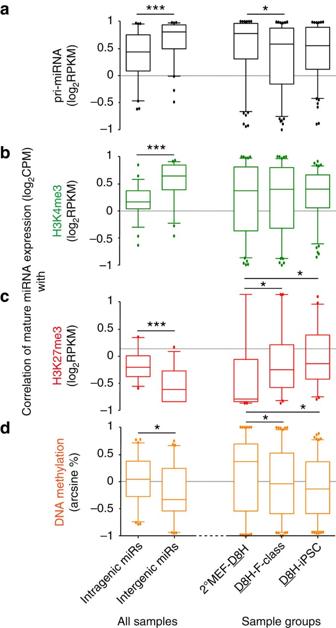Figure 4: Multi-level control of miRNA expression. (a–d) Pearson’s correlation of mature miRNA expression across sample groups and miRNA loci with (a) pri-miRNA expression; (b) promoter H3K4me3; (c) promoter H3K27me3 and (d) promoter DNA methylation4,6. Analysis of pri-miRNA and epigenetic regulation was confined to mature miRNAs fromFigure 3cwhere pri-miRNA levels were detectable and the locus expressing the mature miRNA was unambiguous (128 miRNAs arising from 71 loci). Transcriptional start sites were determined from the 5′ end of observed pri-miRNA. Sample groups are 2°MEFs-D8H (inclusive), D8H-D18H (inclusive) or D8H-iPSC (including D8H, D16L, D21L, D21, 2°IPSCs and 1°IPSCs). Whiskers show 5–95% values.P-values were derived from a two-tailed, heteroscedastict-test (key: *P<0.05 and ***P<0.0001). Related heatmaps are shown inSupplementary Fig. 9. Figure 4: Multi-level control of miRNA expression. ( a – d ) Pearson’s correlation of mature miRNA expression across sample groups and miRNA loci with ( a ) pri-miRNA expression; ( b ) promoter H3K4me3; ( c ) promoter H3K27me3 and ( d ) promoter DNA methylation [4] , [6] . Analysis of pri-miRNA and epigenetic regulation was confined to mature miRNAs from Figure 3c where pri-miRNA levels were detectable and the locus expressing the mature miRNA was unambiguous (128 miRNAs arising from 71 loci). Transcriptional start sites were determined from the 5′ end of observed pri-miRNA. Sample groups are 2°MEFs-D8H (inclusive), D8H-D18H (inclusive) or D8H-iPSC (including D8H, D16L, D21L, D21 , 2°IPSCs and 1°IPSCs). Whiskers show 5–95% values. P -values were derived from a two-tailed, heteroscedastic t -test (key: * P <0.05 and *** P <0.0001). Related heatmaps are shown in Supplementary Fig. 9 . Full size image While dynamic changes of epigenetic marks occurred at many individual miRNA loci ( Supplementary Fig. 9a ), global density of H3K4me3 and DNA methylation remained relatively steady over time ( Supplementary Fig. 9b,d ). By contrast, we observed a global reduction of H3K27me3 density during the first 8 days of high OSKM expression, with a gradual recovery at later time points in the trajectories to both the F-class and ESC-like state ( Supplementary Fig. 9c ). To study the correlation of epigenetic marks with miRNA expression we used the D8H sample, embodying a transiently open chromatin state [4] , as a pivot-point to reveal differences between early and late phases of reprogramming. Averaging across all analyzed miRNA loci, we saw an anti-correlation between H3K27me3 density and miRNA expression at all times during reprogramming; this was strongest in the early phase ( Fig. 4c ). H3K4me3 showed a positive correlation with miRNA expression in all three branches of our time course, while DNA methylation displayed an overall lack of correlation ( Fig. 4b,d ). Altogether, these global patterns are consistent with those observed in parallel for protein coding genes [4] , [5] , [6] . They indicate an acute regulation of miRNA expression by rapid and dynamic changes to histone modifications, especially in early reprogramming, with H3K27me3 removal featuring strongly in early transcriptional change. By contrast, DNA methylation/demethylation less commonly regulates overall miRNA expression, but instead consolidates the expression change of specific miRNAs as cells approach pluripotency. The intricate control of expression at different levels is illustrated by the miR-17/92 group of miRNAs, which stimulate cell proliferation and survival [20] . They fall into four different sequence families, which are expressed from distinct chromosomal loci (see schematic in Fig. 5a ) [20] and are induced during reprogramming in a Myc-dependent manner [21] . Overexpression of miR-106b or miR-93 was furthermore reported to augment OSK-induced reprogramming [21] . Here expression of miRNAs from the miR-92b, miR-106b/25 and miR-17/92 loci was induced early in high OSKM, but receded again upon shift to low OSKM ( Fig. 5a ). Expression of the miR-92b pri-miRNA was extremely low, precluding further analysis. The miR-106b/25 pri-miRNA level rose continuously and was highest in ESC-like controls [4] , indicating prominent transcriptional regulation of this locus towards the F-class state, which is overridden by post-transcriptional controls operating in the ESC-like state. For the miR-17/92 locus, we found multiple active promoters, with one showing selective activity in F-class cells ( Supplementary Fig. 11 ), and possibly giving rise to a pri-miRNA that is more efficiently processed into mature miRNAs, thus explaining the selective accumulation of miR-17/92 miRNAs in this pluripotent state. By contrast, miRNAs from the miR-106a/363 locus correlated well with pri-miRNA expression at all stages ( Fig. 5a ). Transcription at this locus was repressed throughout high OSKM expression but activated as cells progressed towards the ESC-like state. Early loss of H3K27me3 and a transient gain of H3K4me3 were counteracted by an emerging DNA methylation barrier at this promoter, which remained in place in F-class cells. The shift to low OSKM allowed the removal of this barrier and expression of miR-106a/363 in the ESC-like state ( Supplementary Fig. 11 ). These observations shed further light on the complex interplay between transcriptional and post-transcriptional regulation of these loci [22] . Importantly, these data demonstrate that F-class and ESC-like cells acquire equivalent sets of the miR-17/92 group miRNAs, albeit by enhancing the expression of different chromosomal loci. 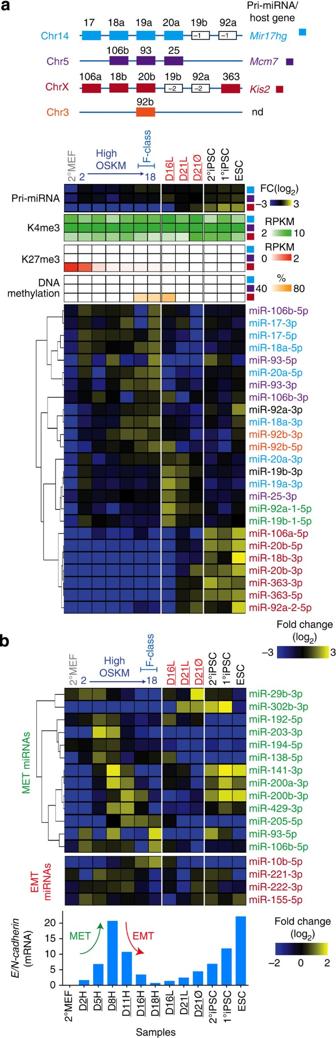Figure 5: Complex regulation of physical loci and functionally related sets of miRNAs. (a) Top: genomic arrangement of miR-17/92a, miR-106b/25, miR-106a/363 and miR-92b loci (boxes outlined in black, loci express identical mature miRNA; nd, pri-miRNA transcript not defined). Middle: expression of pri-miRNAs and epigenetic marks at the respective promoters. Bottom: clustered expression of encoded miRNAs (threshold: >25 counts per million (CPM) average expression per sample). miRNA names are colour-coded by chromosome of origin: Chr 14, green; Chr X, red; Chr5, purple and Chr3, orange. (b) Top: clustered expression of selected pro-MET (green) and pro-EMT miRNAs (red). miRNAs included have defined functions in EMT/MET23,24(threshold: >25 CPM average expression per sample). Bottom; ratio ofE/N-cadherinmRNA expression as a marker of MET/EMT25. Figure 5: Complex regulation of physical loci and functionally related sets of miRNAs. ( a ) Top: genomic arrangement of miR-17/92a, miR-106b/25, miR-106a/363 and miR-92b loci (boxes outlined in black, loci express identical mature miRNA; nd, pri-miRNA transcript not defined). Middle: expression of pri-miRNAs and epigenetic marks at the respective promoters. Bottom: clustered expression of encoded miRNAs (threshold: >25 counts per million (CPM) average expression per sample). miRNA names are colour-coded by chromosome of origin: Chr 14, green; Chr X, red; Chr5, purple and Chr3, orange. ( b ) Top: clustered expression of selected pro-MET (green) and pro-EMT miRNAs (red). miRNAs included have defined functions in EMT/MET [23] , [24] (threshold: >25 CPM average expression per sample). Bottom; ratio of E/N-cadherin mRNA expression as a marker of MET/EMT [25] . Full size image To further explore the complex temporal coordination of cellular processes throughout reprogramming, we analyzed expression patterns of miRNAs involved in the transition between mesenchymal and epithelial cell characteristics (mesenchymal to epithelial transition or epithelial to mesenchymal transition (MET or EMT)) ( Fig. 5b ). This revealed strong but transient increase in pro-MET miRNAs (for example, from the miR-192/194 locus and the miR-200 family), although pro-EMT miRNAs were also induced (for example, from the miR-222/221 locus). The highest expression of pro-MET miRNAs coincided with a peak in E- to N-cadherin ratio and other mesenchymal markers [5] at day 8. Receding expression of pro-MET miRNAs correlated with re-emergence of mesenchymal characteristics in both, high and low OSKM conditions. Notably, F-class cells exhibit a more mesenchymal morphology [3] . This correlated with a much higher expression of the pro-mesenchymal miR-10b-5p [23] and a reduced expression of the pro-epithelial miR-200 family ( Fig. 5b ) and miR-302 locus [23] , [24] in the F-class state. Altogether, these findings are consistent with an initial MET followed by a partial EMT during reprogramming [15] , [25] and they indicate that sequential and pluripotency state-specific changes to the miRNA milieu are involved in promoting these transitions. Distinct miRNA milieus in alternate pluripotent states Next, to focus on differences between the pluripotent states, we compared averaged data from D16H&D18H with 1°iPSCs and 2°iPSCs. This identified 67 miRNAs with greater than fourfold difference between the two groups: 24 were higher in F-class and 43 were higher in ESC-like cells ( Fig. 6a ). Expression differences for miR-378-3p, -205-5p, -10b-5p -21-5p, -302d-3p and -291a-3p were validated by qPCR ( Supplementary Fig. 6 ). We further sequenced the small RNA population of an independently generated F-class clonal cell line (clone 1 day 30 (ref. 3 )), and hierarchical clustering demonstrated that the high OSKM trajectory closely resembled the F-class type in expression of these miRNAs ( Supplementary Fig. 12a ), independently confirming analyses based on mRNA data [3] . 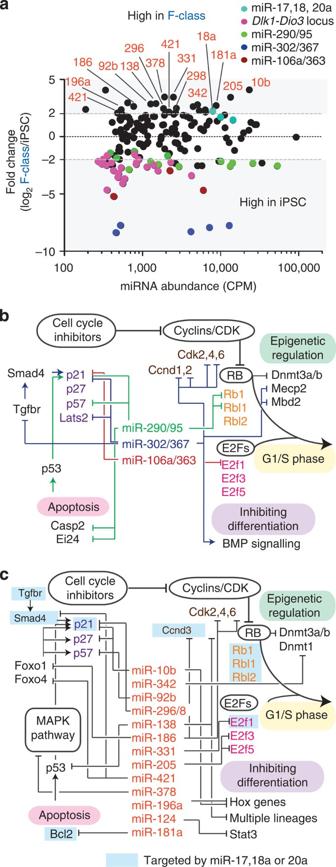Figure 6: miRNA expression distinguishes F-class and ESC-like pluripotency states. (a) Pairwise comparison F-class (average of D16H and D18H) versus iPSC controls (2°iPSC and 1°iPSC) using the 217 miRNAs within the top 95th expression percentile in at least one sample. Fold-change is plotted against average miRNA abundance of the four samples analyzed. miRNA families with known pluripotency roles are denoted by coloured dots: miR-302/367 (dark blue), miR-290/95 (green),Dlk1-Dio3locus miRNAs (pink), miR-106a/363 cluster (dark red), and miR-17, 18 and 20a (light blue). miRNAs listed incare also labelled. (b,c) Diagrams of experimentally verified miRNA/mRNA targeting interactions within pluripotency-related pathways11for miRNAs characteristic of (b) the ESC-like state and (c) the F-class state. Figure 6: miRNA expression distinguishes F-class and ESC-like pluripotency states. ( a ) Pairwise comparison F-class (average of D16H and D18H) versus iPSC controls (2°iPSC and 1°iPSC) using the 217 miRNAs within the top 95th expression percentile in at least one sample. Fold-change is plotted against average miRNA abundance of the four samples analyzed. miRNA families with known pluripotency roles are denoted by coloured dots: miR-302/367 (dark blue), miR-290/95 (green), Dlk1-Dio3 locus miRNAs (pink), miR-106a/363 cluster (dark red), and miR-17, 18 and 20a (light blue). miRNAs listed in c are also labelled. ( b , c ) Diagrams of experimentally verified miRNA/mRNA targeting interactions within pluripotency-related pathways [11] for miRNAs characteristic of ( b ) the ESC-like state and ( c ) the F-class state. Full size image Many miRNAs with higher expression in the ESC-like state have been shown to support pluripotency ( Fig. 6b ) [11] . miRNAs from the imprinted Dlk1 - Dio3 locus, which have context specific cell-cycle, survival and pluripotency functions [12] , [26] , were rapidly downregulated in high OSKM conditions but recovered expression in the low OSKM trajectory and ESC-like controls ( Fig. 3c , cluster I). Expression from the miR-302/367 locus, known to stimulate iPSC cell proliferation, survival, MET and DNA demethylation, was only induced in the low OSKM trajectory and ESC-like controls ( Fig. 3c , cluster A). The ESC-specific miR-290/295 locus, involved in stimulating cell proliferation and survival [11] , gradually increased along both trajectories, but reached its highest level in the fully established ESC-like cell lines ( Fig. 3c , cluster D). Altogether, 12 genomic loci accounted for expression of the ESC-like identifier miRNAs. Eleven of these loci had measurable levels of pri-miRNA transcripts in long RNA-seq data [4] , which correlated well with the expression of the mature miRNAs in seven cases (>0.6 Pearson’s correlation, Supplementary Fig. 12b,c ). Common to both pluripotent states and consistent with an early induction of proliferation during reprogramming [1] , [5] , miRNA levels from the stem cell and placenta-specific miR-466/467/699/297 locus, which promote growth and survival [27] , rapidly rose ( Fig. 3c , cluster E), while those from the anti-reprogramming miR-143/145 locus [12] rapidly declined ( Fig. 3c , cluster J and I). The 24 miRNAs with higher expression in the F-class state were induced by day 2–8 during high OSKM reprogramming, with the notable exception of some let-7 family members (let-7b-5p, let-7-d-5p and let-7-c-5p/miR-99a-5p), miR-196a-5p and 181a-5p, which were maintained at 2°MEF expression level. The switch to low OSKM triggered their downregulation ( Supplementary Fig. 12a and Fig. 3c , cluster B). These miRNAs were derived from 22 genomic loci, 17 of which had measurable pri-miRNA expression. Of these, mature miRNA and pri-miRNA levels were well-correlated for seven loci ( Supplementary Fig. 12b,c ). Analysis of histone and DNA methylation at promoters of F-class and ESC-state identifier miRNAs was often consistent with pri-miRNA expression ( Supplementary Fig. 12b ). Notably, higher expression in the ESC-like state, of the Dlk1 - Dio3 , mir-290/295, miR-106a/363 and miR-302/367 loci, together accounting for 34 of the 43 ESC-like identifiers miRNAs, correlated with loss of DNA methylation, as seen for many ESC-related protein-coding genes [4] , [6] . Altogether, this suggested that epigenetic/transcriptional regulation played a major role in the expression of the ESC-like state identifier miRNAs, with DNA demethylation removing a barrier to their expression late in reprogramming. By contrast, F-class identifier miRNAs were more overtly regulated at the post-transcriptional level. Notable exceptions were miR-10b-5p and 205-5p, whose expression strongly correlated with their respective pri-miRNAs. Repression of these two loci in the ESC-like state appeared to be primarily driven by increased DNA methylation ( Supplementary Fig. 12b ). To assess whether the miRNA milieu of F-class cells can support pluripotency, we analyzed a set of experimentally verified mRNA targets for the F-class identifier miRNAs. Five of the 24 F-class identifier miRNAs had insufficient target information (miR-505, miR-361, miR-1983, miR-301b and miR-652), while four were pro-differentiation let-7 members—let-7b-5p, let-7-d-5p and let-7-c-5p/miR-99a-5p [11] . Nevertheless, other let-7 family members (let-7e-5p, let-7f-5p and let-7g-5p) were downregulated along the trajectories to both F-class and ESC-like states. Remarkably, the targets of 15 F-class identifier miRNAs, although less well-studied in this context, can be grouped into an alternate pro-pluripotency regulatory network ( Fig. 6c ), particularly through targeting self-renewal and cell-cycle pathways (miR-10b-5p, -92b-3p, -296-5p, -298-5p, -138-5p, -186-5p, -331-3p, -205-5p, -421-3p, -18a-5p and -378-3p (through MAPK signalling)). miR-342-3p (ref. 28 ) targets DNA methylation. miR-138-5p (ref. 29 ), miR-196a-5p (ref. 30 ), miR-124-3p (ref. 31 ) and miR-10b-5p (ref. 32 ) are known to inhibit differentiation; importantly miR-138 has recently been shown to promote iPSC generation [29] . miR-181a-5p (ref. 33 ) and miR-18a-5p (ref. 20 ) (also miR-17 and -20a) promote cell survival ( Fig. 6c ). Thus, the deficiency of F-class cells in well-characterized pluripotency-associated miRNAs can be compensated for by higher expression of another functionally equivalent subset. In further support of the relevance of both ESC-like and F-class identifier miRNAs we found that their levels and those of proteins encoded by their validated mRNA targets showed substantial co-dependence during reprogramming ( Supplementary Fig. 12d ). As expected, most cases exhibited inverse correlation. Interestingly, in the F-class state, several targets showed positive correlation with their corresponding miRNA. Co-regulation by OSKM transcription factors, of miRNAs as well as targets, suggests potential incoherent feed-forward relationships in these cases [34] . Altogether, we present here the most comprehensive small RNA expression analysis of somatic cell reprogramming to date, featuring high temporal resolution, as well as nucleotide level precision to reveal complex patterns of regulated miRNA biogenesis to support distinct states of cellular pluripotency. Together with the concordant long RNA transcriptome, global proteome and CpG methylation data [4] , [5] , [6] , this work provides a unique resource to study dynamic genome expression during iPSC generation. Sample preparations for small RNA sequencing Murine Rosa26-rtTA knock-in ESCs [35] , 1°IPSCs, 2°IPSCs (1B system) [36] and 2°MEFs were cultured as previously described [37] . Reprograming of 2°MEFs was induced by exposure to doxycycline in the media using methods described in the study by Hussein et al . [4] Duration and concentration of doxycycline treatments as well as the sampling strategy are detailed in Fig. 1a and cells were harvested for RNA extraction at the indicated times. Specifically, 13 sequencing libraries were initially sequenced, derived from: 1°IPSCs, 2°IPSCs, ESCs, 2°MEFs; high-dox treated cells (1,500 ng ml −1 doxycycline) at day 2, 5, 8, 16 and 18; low-dox treated cells (1,500 ng ml −1 for 8 days, then 5 ng ml −1 )) at day 16 and 21 (D16L and D21L, red circles); and low-dox treated cells (1,500 ng ml −1 for 8 days, 5 ng ml −1 doxycycline for 6 days and then no doxycycline) at day 21 (D21 ). To gain greater resolution of early changes, five further libraries were subsequently sequenced from the same experiment: 2°MEFs and high-dox treated cells (1,500 ng ml −1 doxycycline) at days 1, 2, 3 and 4. For comparison to the described F-class state [3] , a small RNA library was also created from an independently generated F-class clone (clone 1, day 30). RNA was extracted from cells using the mirVana miRNA isolation kit (Ambion) following the manufacturer’s instructions. Small RNA libraries for NGS were prepared using the small RNA preparation protocol of the SOLiD Total RNA-Seq kit as per the manufacturer’s instructions. Specifically, size selection was performed to include RNA between 18–38 nt in length. Library sequencing was either performed on a SOLiD version 4 (samples of the high/low OSKM trajectories: 2°MEF, D2H, D5H, D8H, D11H, D16H, D18H, D16L, D21L, D21 , 1°iPSC, 2°iPSC and ESC) or a SOLiD 5500 NGS instrument (samples from the day 0–4 high OSKM time course: 2°MEF E , D1H E , D2H E , D3H E , D4H E and F-class clone 1, day 30). Mapping of NGS data We refer to an individual NGS read as a tag and the number of times it occurred as a tag count. Prior to mapping, a custom Perl script was used to trim adapters from the sequence tags and remove all tags with an average quality value of <18 across the tag ( Supplementary Software 1 ). In addition, all tags containing ambiguous colour calls represented by ‘.’ were also removed from further analysis. The remaining high quality tags were then mapped to the male mouse genome reference (assembly version mm9, 18S rRNA gi|374088232 and 28S rRNA gi|120444900) by using Bowtie software [38] , version 0.12.8, that supports colour-space data mapping ( Supplementary Software 2 ). Mapping parameters were chosen such that up to two colour-space mismatches were allowed in the first 20-nt seed region, and alignment was extended to the full-length of the tag if the sum of the quality values at mismatch positions did not exceed 70. Full mapping details and miRNA variant analysis are described in the Supplementary Methods and data found in Supplementary Data 1 and 2 . Individual miRNA variants for each sequenced sample can be visualized in associated miRspring [19] documents, Supplementary Data 3–21 . Clustering and differential expression analysis For clustering and PCA, only miRNAs in the 95th percentile of expression in at least one library were used, and their expression was normalized to their average expression and log 2 transformed. Principal component analysis was performed using Multi Experiment Viewer v4.8 ( http://mev-tm4.sourceforge.net/ ) [39] . For the core samples, clustering was performed using Pearson's correlation and complete linkage with 10,000 rounds of boostrapping to generate approximate unbiased test scores. Scores above 60% were considered significant and discrete clusters were generated from the first node where this threshold was met ( Supplementary Fig. 7 ). Other clustering was performed using Pearsons correlation and complete linkage with 10,000 rounds of bootstrapping without discrete clustering based on unbiased test scores using Multiple Experiment Viewer v4.8 ( Supplementary Figs 8 and 12 ). Pairwise comparisons were restricted to miRNAs in the top 95% of tags in at least one of the samples being compared with a fourfold threshold. The comparisons were run with edgeR [40] . miRNA target and GO analysis Experimentally verified vertebrate targets of all vertebrate miRNAs were downloaded from miRtarbase [41] . GO and pathway enrichment analysis were performed using DAVID [42] with the total list of known miRNA-targeted mRNAs as the background. Significant enrichment was defined as P <0.01 for biological processes and P <0.05 for molecular function, cellular component and KEGG pathways (Benjamini–Hochberg P-values corrected for multiple testing). Target predictions were made using customized TargetScan code [43] to determine all potential seven-mer and eight-mer seed sites (irrespective of conservation or context scores) in Ensembl transcripts determined as expressed above the level of background noise by the Alexa-seq [44] analysis of RNA-seq data [4] . For correlation of expression of known protein targets of miRNAs, log 2 -transformed protein expression data were Pearson’s correlated with log 2 -transformed miRNA expression data. To generate a random background of miRNA:protein correlations, >10,000 random miRNA and protein combinations were created using miRNAs expressed in the top 95th percentile of expression in at least one sample analyzed and proteins with complete data for all samples analyzed. Quantitative PCR qPCR detection was based on methods published previously [45] and primer sequences are listed in Supplementary Data 1 . Reverse transcription (RT) was carried out accordingly with the TaqMan miRNA Reverse Transcription Kit (Life Technologies). For each PCR reaction: 2 μl of 10 × diluted RT product was added to 10 μl of LuminoCt SYBR Green qPCR ReadyMix (Sigma) along with 10 pmol of each qPCR primer and ddH 2 O up to 20 μl. miRNAs were quantified using the CFX96 Real-Time Detection System (Bio-Rad); qPCR conditions were: 95 °C for 10 s, 58 °C for 8 s; × 40 cycles. Validation of miR-292-3p target sites in Clock miRNA target validation using dual luciferase assay was performed as previously described [46] . Specifically, two regions of the Clock 3′ untranslated region (UTR) containing putative binding sites of miR-292-3p (~500 bp each) were each amplified by PCR from C57Bl/6 mouse genomic DNA using Platinum Taq polymerase (Life Technologies) and cloned into the pGEM-T-Easy (Promega) ‘TA’-cloning vector for sequence verification. Mutant plasmids were generated by amplifying the pGEM-T plasmids containing putative mir-292-3p sequences using Phusion proof-reading Polymerase (Finnzyme). The seed regions of the putative mir-292-3p miRNA binding sites were mutated using primers incorporating SbfI restriction enzyme sites. This was done using by PCR amplification of the whole template using 5′-end phosphorylated primers and the resultant PCR product ligated. Primer sequences are as follows: mCLOCK 3′ UTR Site 1 WT Forward (F), 5′- AAC AAT GTG CTG CTG GGA AT -3′; mCLOCK 3′ UTR Site 1 WT Reverse (R), 5′- TCA TGG GGA CTT GAG AAT GA -3′; mCLOCK 3′ UTR Site 1 WT F, 5′- CAA GCC TTA GAA AGG ACC CTT AG -3′; mCLOCK 3′ UTR Site 1 WT R, 5′- GCA GAA GGG GAG GGA ATT AG -3′; mCLOCK 3′UTR Site1 mut F, 5′- TTT TAA CAT TCT CAG AGG TGG GAA T -3′; mCLOCK 3′UTR Site1 mut R, 5′- CCT GCA GGT AAA ATG TTT TGT GTG CAA -3′; mCLOCK 3′UTR Site2 mut F, 5′- GCC ATT TTC ATA GTG ATT GCA TAA AGA -3′; mCLOCK 3′UTR Site2 mut R, 5′- CCT GCA GGT TGT GCT GTT TCT TCA CC -3′. The sequence-confirmed wild-type and mutant 3′ UTR sequences were each excised from pGEM-T-Easy vector and inserted into the NotI site of pSiCHECK2 vector (Promega) downstream of the Renilla luciferase gene. This vector also contains a firefly luciferase gene to normalize for transfection efficiency. Synthetic miRNA mimics mouse miR-292-3p (Cat# C310472-05-00005), and negative control (cel-miR-67, Cat# CN-001000-01-05) were purchased from ThermoFisher Scientific, Lafayette, CO, USA. NIH-3T3 cells were maintained in DMEM supplemented with 10% (v/v) foetal calf serum and antibiotics. Cells were plated at 1 × 10 4 cells per well in a 96-well plate 1 day prior to transfection, at which point they had reached 80–90% confluency. The cells were co-transfected with the pSiCHECK2 plasmid containing the desired insert (100 ng) and the miRNA mimic (100 nM) using DharmaFECT Duo Transfection Reagent (ThermoFisher Scientific). Firefly and Renilla luciferase activity was measured consecutively using a Dual Luciferase Assay Kit (Promega) 24 h after transfection using a PolarStar luminometer and plate reader (BMG Labtech). Promoter histone and DNA methylation analysis miRNA transcriptional start sites (TSS) were annotated from the 5′-ends of observed pri-miRNAs defined as a continuous transcript overlapping the miRNA hairpin observed in the long RNA sequencing [4] . H3K4me3, H3K27me3 and H3K36me3 read density around TSSs, as well as percentage of DNA methylation, were measured from data described in refs 4 . Specifically, histone trimethylation measurements were restricted to −2 and+3 kb around TSS. DNA methylation measurements were restricted to −1 and +1 kb. In addition, for the Dlk1 - Dio3 locus we analyzed previously reported IG-DMR coordinates [47] . Correlation of mature miRNA expression with pri-miRNA and H3 methylation was performed on log 2 -transformed RPKM/counts per million with Pearson’s correlation. Pearson’s correlation of mature miRNA expression was performed using arcsine-transformed percentage of DNA methylation and log 2 -transformed miRNA expression (counts per million). P -values were determined using a two-tailed, heteroscedastic t -test. Long RNA sequencing was performed as described in the study by Hussein et al . [4] Histone methylation ChIP and DNA methylation sequencing was performed as described in refs 4 , 6 . How to cite this article : Clancy, J. L. et al . Small RNA changes en route to distinct cellular states of induced pluripotency. Nat. Commun. 5:5522 doi: 10.1038/ncomms6522 (2014). Accession codes: Small RNA, long RNA and Chip-Seq raw data have been deposited in the NCBI Sequence Read Archive (SRA) under the accession code SRP046744 . Methylome sequencing data are available from the European Nucleotide Archive (ENA) under accession code ERP004116 ( http://www.ebi.ac.uk/ena/data/view/PRJEB4795 ). Proteomics data have been deposited in the ProteomeXchange under accession code PXD000413. Processed data and visualization options through the UCSC browser are further available at the Project Grandiose web portal ( http://www.stemformatics.org/projects/project_grandiose ).